Antarctic contribution to meltwater pulse 1A from reduced Southern Ocean overturning During the last glacial termination, the upwelling strength of the southern polar limb of the Atlantic Meridional Overturning Circulation varied, changing the ventilation and stratification of the high-latitude Southern Ocean. During the same period, at least two phases of abrupt global sea-level rise—meltwater pulses—took place. Although the timing and magnitude of these events have become better constrained, a causal link between ocean stratification, the meltwater pulses and accelerated ice loss from Antarctica has not been proven. Here we simulate Antarctic ice sheet evolution over the last 25 kyr using a data-constrained ice-sheet model forced by changes in Southern Ocean temperature from an Earth system model. Results reveal several episodes of accelerated ice-sheet recession, the largest being coincident with meltwater pulse 1A. This resulted from reduced Southern Ocean overturning following Heinrich Event 1, when warmer subsurface water thermally eroded grounded marine-based ice and instigated a positive feedback that further accelerated ice-sheet retreat. Geologically constrained numerical model simulations indicate that during the last glacial termination (T1, 19–11 ka before present (BP)) the Antarctic ice sheets (AIS) contributed 10–18 m to global mean sea level (GMSL) rise [1] , [2] , [3] , [4] , [5] . However, whether the AIS made a substantial contribution to deglacial meltwater pulses is still a matter of debate, as a well-constrained quantitative estimate of the volume, timing and rate of freshwater flux from the AIS is still lacking. For Antarctica to have made a meaningful contribution to deglacial meltwater pulses (MWP1A and MWP1B) during T1 (hereafter referred to as the ‘AIS MWP theory’), three conditions must be satisfied. First, sufficient sea-level equivalent (s.l.e.) ice volume must have existed in Antarctica at the Last Glacial Maximum (LGM). Second, this ice volume must have been discharged at the correct time and at a fast-enough rate to contribute to the rapid rises in sea level. Third, a plausible mechanism must exist by which the previous two conditions are met. Here we present a suite of ice-sheet modelling experiments that employ a range of proxy-based and modelled sea level and ocean temperature time series to generate a suite of possible Antarctic ice-sheet retreat scenarios. Our simulations use the latest sea-level reconstruction from Tahiti [6] , the most probable (centreline) scenario from a probabilistic assessment of six far-field sea-level records [7] , and from a glacio-isostatic adjustment model simulation of eustatic sea level [8] ( Supplementary Fig. 1a ). We combine each of these with each of four scenarios representing changes in ocean heat through T1, from a global stack of 57 deep-ocean records [9] , a Southern Ocean-specific record from offshore New Zealand [10] and from two transient simulations of the last deglaciation using an intermediate complexity Earth System model—one that incorporates a high southern latitude freshwater input (freshwater forcing (FWF)) at the time of MWP1A, and one that does not (no freshwater forcing (NFW)) [11] ( Supplementary Fig. 1b ). As the two Earth System model simulations differ only in the prescription (or not) of a Southern Ocean freshwater flux, we are able to use these two scenarios to isolate the differences in ice-sheet response that arise solely as a consequence of this forcing. Other than the different sea level and ocean heat forcings, all of the deglacial simulations use identical glaciological parameterization, time-dependent air temperature and precipitation forcings, as well as an isostatic model. Based on the ensemble mean, the simulations reveal that centennial-scale periods of accelerated ice mass loss could have occurred during the last glacial termination, with the largest such event coinciding with MWP1A. However, for the AIS to have contributed substantially to this event we find that a specific interaction between the ice sheet and its surrounding ocean is necessary. Specifically, mass loss rates are highest when an abrupt reduction in Southern Ocean overturning allows rapid subsurface oceanic warming to take place. Fit to LGM ice extent To produce an ice-sheet geometry that closely agrees with ice-core interpretations of LGM surface elevation changes and marine geological reconstructions of LGM extent, and reproduces the pattern of temporal evolution in each sector of the ice sheet, we ran a suite of simulations representing a range of glaciological parameterizations. Outputs from each experiment were assessed against a range of empirical constraints to gauge overall closeness-of-fit (see Methods). The simulation considered to reflect the ‘best-fit’ to these constraints is shown in Fig. 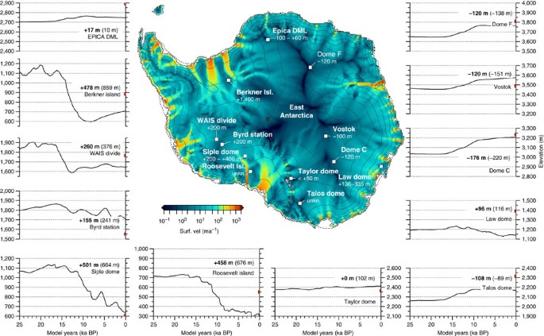Figure 1: Geometry and dynamics of the ensemble mean LGM AIS. Main panel shows locations of ice cores used for constraint and their interpreted LGM elevation or thickness change from present. Geologically interpreted LGM grounding-line positions shown with dashed line18. Marginal panels show time series of modelled surface elevation changes at each of the ice core sites. Simulated LGM to present-day elevation change and thickness at each ice core site are shown in bold and parenthesis respectively. ‘LGM’ in this case is defined as the maximum elevation/thickness reached during the period 25–20 ka BP, thus may not be contemporaneous between sites. Red squares denote present-day ice-sheet surface elevations. 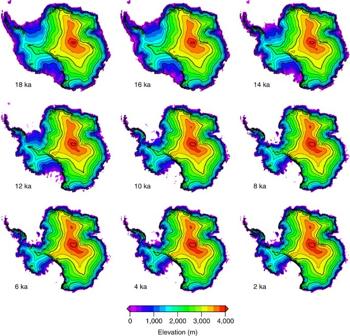Figure 2: Time slices of AIS extent through T1. Panels show mean surface elevations from the model ensemble. Note the lowering of East Antarctica, thickening in West Antarctica and lateral expansion around the entire continent at LGM. Grounding lines achieve a position close to present-day locations by 6–8 ka BP. 1 , based on the parameterization described in Supplementary Table 1 and the ice-core constraints listed in Supplementary Table 2 . The pattern of LGM thickening with respect to modelled present-day ice thickness is robustly captured at most sites, although the model underestimates absolute present-day elevations at Law Dome by ~18%. In general, mismatches in modelled versus observed surface elevation at the end of the model run are most pronounced on coastal islands, such as Law Dome, Berkner Island and Roosevelt Island. Model-data fit is far better in continental interior areas such as Dome F (<1% difference in elevation), Vostok (<3%), Dome C (<1%) and the West Antarctic Ice Sheet (WAIS) Divide (<6%). This gives us confidence that the ice-sheet model is performing reliably, and we attribute the peripheral mismatches primarily to unintended consequences of the spin-up procedure, principally the initial smoothing run that relaxes the ice surface from its initial state to one that is slightly smoothed. Figure 1: Geometry and dynamics of the ensemble mean LGM AIS. Main panel shows locations of ice cores used for constraint and their interpreted LGM elevation or thickness change from present. Geologically interpreted LGM grounding-line positions shown with dashed line [18] . Marginal panels show time series of modelled surface elevation changes at each of the ice core sites. Simulated LGM to present-day elevation change and thickness at each ice core site are shown in bold and parenthesis respectively. ‘LGM’ in this case is defined as the maximum elevation/thickness reached during the period 25–20 ka BP, thus may not be contemporaneous between sites. Red squares denote present-day ice-sheet surface elevations. Full size image Comparison with present-day ice sheet At the end of the simulation, our model runs closely replicate present-day ice-sheet geometry and surface velocity field ( Supplementary Fig. 2 ). In particular, the ensemble mean predicts a present-day grounded-ice volume that is within 2% of the modern volume [12] , and reproduces the locations, flow speeds and drainage patterns of discrete ice streams around the margins of the ice sheet. This check ensures not only that the glaciological parameterization is well-tuned, but also that the transient forcings are appropriately scaled. For comparison with measured bedrock uplift rates around the continent, we extract the pattern and magnitude of the ongoing rebound signal from the final time slice of our model. Residual uplift maxima lie in the inner Weddell and Ross seas, with lower rates around most of the modern coastline and across most of the Antarctic Peninsula. Bedrock elevation change is close to zero for interior East Antarctica and central WAIS, with slow subsidence modelled in some sectors ( Supplementary Fig. 3 ). Despite considerable uncertainties in the Global Positioning System (GPS)-derived data, the overall pattern shown by the model is consistent with the pattern indicated by the available measurements ( Supplementary Fig. 3 ). Evolution of ice-sheet geometry By tuning our model to reproduce both present-day and LGM configurations, we have confidence that the changes simulated between the two end-member states during T1 are robust. Ice-sheet evolution through T1, from the expanded LGM ice sheet at 18 ka BP, through to the present-day configuration, which is more-or-less attained by the mid-Holocene, is illustrated in Fig. 2 . Ice surface elevations in East Antarctica are slightly lower at the LGM than at present, due to declining precipitation under colder, drier, full glacial conditions. These climatic changes also affect West Antarctica, but the surface here rises, in agreement with ice core interpretations. This thickening of the WAIS occurs in response to grounding-line migration in the Ross, Weddell and Amundsen Sea basins, and the increased buttressing that this newly grounded ice provides. As a consequence of net ablation in McMurdo Sound, imposed to allow closer fit to geological data there [13] , [14] , the modelled ice surface in the western Ross Sea slopes northwestward and allows ice flux into the sound from glaciers to the south (primarily Byrd, Mulock and Skelton glaciers). The ensemble mean predicts an LGM ice surface elevation adjacent to the Dry Valleys of 300–450 m above the present sea level. Grounding-line recession in the Ross Sea occurs earliest in the centre of the embayment, with grounded ice persisting along the present-day coastline until the early Holocene. In the Weddell Sea embayment, grounding-line recession occurs earliest in eastern and western troughs, with slower-flowing ice in the central embayment retreating latest ( Fig. 2 ). Figure 2: Time slices of AIS extent through T1. Panels show mean surface elevations from the model ensemble. Note the lowering of East Antarctica, thickening in West Antarctica and lateral expansion around the entire continent at LGM. Grounding lines achieve a position close to present-day locations by 6–8 ka BP. Full size image Ice discharge and contribution to sea level In the experimental ensemble, we use two proxy-based and two model-based time series forcings to control the basal mass balance of ice shelves. The proxy forcings use empirical records that reflect either deep-ocean temperature changes through the last glacial cycle [10] or the combination of ice volume and deep-ocean temperature changes [9] . The former is a Southern Ocean record, whereas the latter is a global stack. Both records, however, show that the fastest warming took place between 18 and 11 ka BP, with evidence in the Southern Ocean proxy [10] of an abrupt deep-ocean warming coincident with MWP1A ( Supplementary Fig. 1b ). Mid-depth temperature trends in our model simulations [11] , [15] reveal more highly resolved changes, but the overall pattern of fastest warming from around 18 to 11 ka BP is consistent with the empirical proxies. Notable deviations from the coarsely resolved proxy records include two abrupt warming events at 16 ka BP and, in our freshwater forcing experiment (FWF), at 14.4–12.8 ka BP. The consequence of these forcings in terms of modelled ice-sheet volume response is shown in Fig. 3 . Taking the ensemble mean, Fig. 3a shows that the maximum ice volume of the LGM AIS reaches 32.3 × 10 6 km 3 by 20 ka BP, ~5.8 × 10 6 km 3 greater than that of the modern ice sheet [12] . This represents a eustatic s.l.e. lowering of ~14.5 m. Isostatic subsidence, however, as well as the replacement of ocean with grounded ice in some areas, means that the isochronous sea-level relevant ice volume is closer to 10.5 m. Simulations using the Southern Ocean proxy [10] produce peak mass loss rates during T1 of 1.5–2.5 mm per year s.l.e. (2.5–4 mm per year uncorrected for isostatic loading and density changes) at 14.5 and 12 ka BP, whereas the global proxy [9] leads to a maximum discharge rate of around 1.5–2 mm per year s.l.e. (2–3 mm per year uncorrected) at 14.2, 13 and 11.5–8.9 ka BP. Simulations forced with modelled temperatures from the FWF experiment produce a short-lived discharge pulse of up to 6.7 mm per year s.l.e. (10.5 mm per year uncorrected) at 14.4 ka BP and a secondary, broader peak that averages around 1–2 mm per year s.l.e. (3–4.5 mm per year uncorrected) at 11.5–10.5 ka BP. By contrast, the NFW simulations yield greatest mass loss (2–3.5 mm per year s.l.e., 5–6 mm per year uncorrected) only during this later phase (11.5–10.5 ka BP). 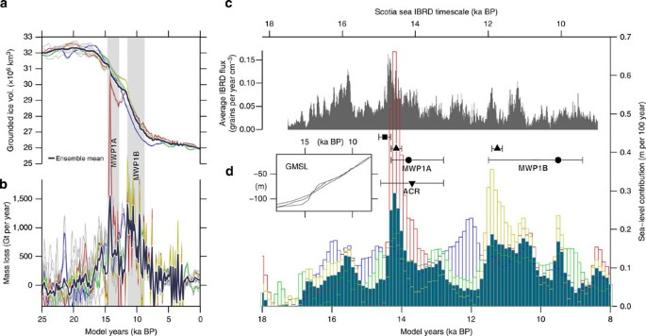Figure 3: Ice volume and sea-level contributions of the LGM AIS. (a) Modelled ice volume time series from the LGM through to present, from the ensemble simulations using three sea-level6,7,8and four ocean temperature reconstructions. Grey lines show individual experiments, coloured lines denote means of each set of ocean temperature forcings (blue10, green9, FWF, red11and NFW, yellow11), dark line shows ensemble mean. (b) Simulated rates of ice-sheet mass loss, colour scheme same as above. Grey shading denotes maximum temporal envelope of meltwater pulses 1A and 1B6,7,63. (c) Iceberg-rafted debris variability in the Scotia Sea during the period 18–8 ka BP16. Note the slightly different timescale compared withd. (d) Simulated sea-level contribution through the period 18–8 ka BP, binned at 100-year intervals, for group means and ensemble mean (solid blue). Timings of meltwater pulses 1A and 1B shown with error bars reflecting probable duration, from ref.6(square), ref.63(triangle) and ref.7(circle). Inset shows GMSL through this interval6,7,8. Figure 3: Ice volume and sea-level contributions of the LGM AIS. ( a ) Modelled ice volume time series from the LGM through to present, from the ensemble simulations using three sea-level [6] , [7] , [8] and four ocean temperature reconstructions. Grey lines show individual experiments, coloured lines denote means of each set of ocean temperature forcings (blue [10] , green [9] , FWF, red [11] and NFW, yellow [11] ), dark line shows ensemble mean. ( b ) Simulated rates of ice-sheet mass loss, colour scheme same as above. Grey shading denotes maximum temporal envelope of meltwater pulses 1A and 1B [6] , [7] , [63] . ( c ) Iceberg-rafted debris variability in the Scotia Sea during the period 18–8 ka BP [16] . Note the slightly different timescale compared with d . ( d ) Simulated sea-level contribution through the period 18–8 ka BP, binned at 100-year intervals, for group means and ensemble mean (solid blue). Timings of meltwater pulses 1A and 1B shown with error bars reflecting probable duration, from ref. 6 (square), ref. 63 (triangle) and ref. 7 (circle). Inset shows GMSL through this interval [6] , [7] , [8] . Full size image Overall, the ensemble mean shows rapid mass loss between 16.5 and 8.5 ka BP, with fastest rates occurring during two main events at 14.5–14 and 11.6–10.2 ka BP, and a smaller precursor event at 16.2–15.2 ka BP. Antarctic ice loss appears to almost halt between 13.1 and 11.8 ka BP. The early phase of ice loss, coincident with MWP1A, mostly affects the Antarctic Peninsula and the mid to outer Weddell Sea, with a small amount of thinning and grounding-line retreat also taking place in the central part of the outer Ross Sea ( Fig. 4a,e ). The second, more prolonged period of discharge (synchronous with MWP1B) takes place primarily in the inner parts of the major marine embayments of the Weddell and Ross seas, and along the length of the Amery Trough ( Fig. 4c ). Despite only being constrained to fit LGM and present-day ice-sheet geometries, the ensemble-mean prediction of ice-sheet mass-loss events (‘meltwater pulses’) through the deglacial period ( Fig. 3d ) shows remarkable agreement with a new record of iceberg-rafted debris from the Scotia Sea [16] ( Fig. 3c ). This latter record is based on counts of coarse-grained sediments deposited from icebergs, whereas our simulation of mass loss arises from melting, as we impose no explicit iceberg calving in our model. Nonetheless, allowing for subtle differences in timing, there is a clear correspondence between the two records in terms of the broad chronology and relative magnitudes of ice-sheet change through T1 ( Fig. 3c,d ). 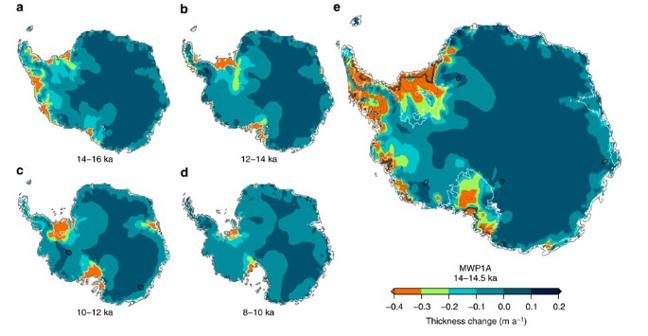Figure 4: Rate of ice mass loss during the period 16–8 ka BP from the ensemble mean simulation. (a) Earliest ice-sheet thinning is greatest around the Antarctic Peninsula and in the outer Weddell Sea; (b) margin retreat continues through 14–12ka BP but (c) the greatest rates of sustained mass loss occur at 12–10 ka BP in the inner Weddell, Ross and Amery embayments. (d) By 8 ka BP modelled grounding lines are close to present-day positions and continuing retreat is slow. (e) During MWP1A (14–14.5 ka BP), fastest ice loss occurs in the Weddell Sea and around the Antarctic Peninsula, with thinning in the Ross Sea largely restricted to the central embayment. Figure 4: Rate of ice mass loss during the period 16–8 ka BP from the ensemble mean simulation. ( a ) Earliest ice-sheet thinning is greatest around the Antarctic Peninsula and in the outer Weddell Sea; ( b ) margin retreat continues through 14–12ka BP but ( c ) the greatest rates of sustained mass loss occur at 12–10 ka BP in the inner Weddell, Ross and Amery embayments. ( d ) By 8 ka BP modelled grounding lines are close to present-day positions and continuing retreat is slow. ( e ) During MWP1A (14–14.5 ka BP), fastest ice loss occurs in the Weddell Sea and around the Antarctic Peninsula, with thinning in the Ross Sea largely restricted to the central embayment. Full size image In summary, the suite of simulations appears to satisfy the first two requirements of the AIS MWP theory. We simulate an ice sheet with sufficient excess ice volume to contribute significantly to deglacial meltwater pulses, and the predicted episodes of fastest mass loss are consistent with the timings of MWP1A and MWP1B. In the ensemble mean, peak rates of mass loss are relatively low (<0.3 m s.l.e. per century), but under our most extreme forcing these rates are more than double, contributing around 2 m s.l.e. over the 350-year timeframe of MWP1A [6] . Assuming a total MWP1A sea-level rise of at least 14 m and a Northern Hemisphere contribution to this of 6.5–10 m [17] , Antarctica and other Southern Hemisphere ice masses presumably contributed to the remaining 4–7.5 m s.l.e. During each of the two broad periods spanning MWP1A (15–13 ka BP) and MWP1B (12–10 ka BP), our simulations suggest ice loss from Antarctica ranging from 1.7 to 4.3 m s.l.e. Sea-level lowering is insufficient to force AIS expansion to the continental shelf edge as inferred from geological data [18] . Thus, cooler ocean temperatures are also required so that ice shelves thicken and become grounded [2] , [3] . This oceanic mass-balance control becomes increasingly important when atmospheric temperatures decline during the LGM, as the colder and drier air masses supply less precipitation to the ice-sheet surface. During T1, these environmental controls reversed. Sea level rose, ocean temperatures increased and atmospheric conditions became warmer and wetter. All of our simulations incorporate these changes, yet only those that are forced with an abrupt increase in ocean temperature at 14.4–12.4 ka BP produce a meltwater ‘pulse’ that is more than double the amplitude of other periods of mass loss ( Fig. 3d ). Abrupt rises in sea level [6] , [8] do not, on their own, trigger rapid retreat of the modelled AIS, nor do rapidly warming air temperatures [19] . Therefore, to satisfy the third requirement of the AIS MWP theory, a valid mechanism must exist by which an abrupt subsurface ocean warming might take place, and by which this warming could subsequently trigger the rapid retreat of grounded ice. Proxy data from Antarctica and the Southern Ocean reveal an abrupt reduction in Southern Ocean upwelling following Heinrich Event 1 (H1), perhaps due to rapid recovery of the Atlantic Meridional Overturning Circulation ( Fig. 5a ) at this time [20] , [21] . Reduced Antarctic Bottom Water (AABW) formation [22] , [23] leads to atmospheric cooling over Antarctica [19] and a reduction in sea-surface temperature over the Southern Ocean [21] , [24] ( Fig. 5c,f )—the Antarctic Cold Reversal. Expansion of sea ice further inhibits ventilation, while the decrease in AABW formation also leads to a subsurface warming in the Southern Ocean ( Fig. 5d ) and close to the Antarctic coast [15] . 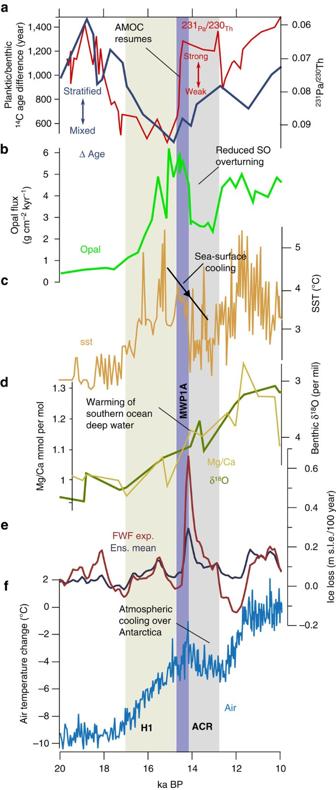Figure 5: Proxy records of oceanic and atmospheric changes during T1. Antarctic and Southern Ocean proxy records of environmental changes; (a) changes in Southern Ocean stratification (blue) from core MD07-3088, 46° S21and Atlantic Meridional Overturning Circulation (AMOC) strength (red) from231Pa/230Th ratios in core GGC5 (ref.20) both in anti-phase with (b) opal flux (green) at 53° S (core TN057-13 (ref.64)), a proxy for upwelling south of the polar front; and (c) diatom-based sea-surface temperature trend from Southern Ocean core TN057-13 (ref.24). (d)δ18O and Mg/Ca deep Southern Ocean temperature proxies from Ocean Drilling Program Leg 118 core MDV-1123 (ref.10); (e) modelled s.l.e. AIS ice mass loss for ensemble mean and the freshwater forcing experiment; and (f) atmospheric cooling during the ACR (Antarctic Cold Reversal) in the EPICA Dome C oxygen isotope record19. H1, Heinrich Event 1; MWP1A, meltwater pulse 1A. Figure 5: Proxy records of oceanic and atmospheric changes during T1. Antarctic and Southern Ocean proxy records of environmental changes; ( a ) changes in Southern Ocean stratification (blue) from core MD07-3088, 46° S [21] and Atlantic Meridional Overturning Circulation (AMOC) strength (red) from 231 Pa/ 230 Th ratios in core GGC5 (ref. 20 ) both in anti-phase with ( b ) opal flux (green) at 53° S (core TN057-13 (ref. 64 )), a proxy for upwelling south of the polar front; and ( c ) diatom-based sea-surface temperature trend from Southern Ocean core TN057-13 (ref. 24 ). ( d ) δ 18 O and Mg/Ca deep Southern Ocean temperature proxies from Ocean Drilling Program Leg 118 core MDV-1123 (ref. 10 ); ( e ) modelled s.l.e. AIS ice mass loss for ensemble mean and the freshwater forcing experiment; and ( f ) atmospheric cooling during the ACR (Antarctic Cold Reversal) in the EPICA Dome C oxygen isotope record [19] . H1, Heinrich Event 1; MWP1A, meltwater pulse 1A. Full size image The Earth System model reproduces the cooler air and sea-surface temperatures of the Antarctic Cold Reversal ( Fig. 6a,b ) as well as the subsurface warming shown in Southern Ocean benthic temperature reconstructions [10] ( Fig. 6c ); yet, for the Southern Ocean to influence the AIS there must be direct connectivity. At the end of H1, AIS grounding lines were close to the continental shelf edge and thus proximal to Circumpolar Deep Water rising up the continental slope ( Fig. 7a ). If the relatively warm Circumpolar Deep Water reached the AIS, it would accelerate ice-sheet melt and further freshen the ocean surface, providing an amplifying feedback ( Fig. 7b ). Increased grounding-line melt brings about ice-shelf thinning, leading to the acceleration of adjacent grounded ice. Longitudinal coupling in this fast-flowing ice transmits the effects of the oceanic perturbation inland from the grounding line, lowering the ice-sheet surface and increasing horizontal fluxes (that is, discharge). Converting this discharge into equivalent freshwater input to the ocean, we simulate a maximum flux of 0.11 Sv (3,950 Gt per year), a value sufficient to shut down AABW formation in the Earth System model [11] . Thus, during MWP1A the modelled ice-sheet response is of sufficient magnitude to maintain oceanic stratification, and promote further ice-sheet retreat. 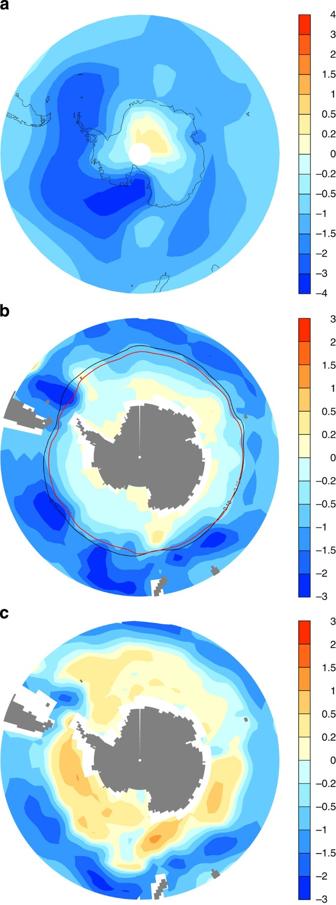Figure 6: Modelled consequence of freshwater input to the Southern Ocean. (a) Surface air temperature anomaly, showing atmospheric cooling (Antarctic Cold Reversal) throughout the southern hemisphere11; (b) sea surface temperature anomaly, also showing the expansion and thickening of sea ice (black line shows extent, red line shows 0.1 m contour); and (c) ocean temperature anomaly at 485–700 m water depth showing pervasive warming of subsurface water around Antarctica. Figure 6: Modelled consequence of freshwater input to the Southern Ocean. ( a ) Surface air temperature anomaly, showing atmospheric cooling (Antarctic Cold Reversal) throughout the southern hemisphere [11] ; ( b ) sea surface temperature anomaly, also showing the expansion and thickening of sea ice (black line shows extent, red line shows 0.1 m contour); and ( c ) ocean temperature anomaly at 485–700 m water depth showing pervasive warming of subsurface water around Antarctica. 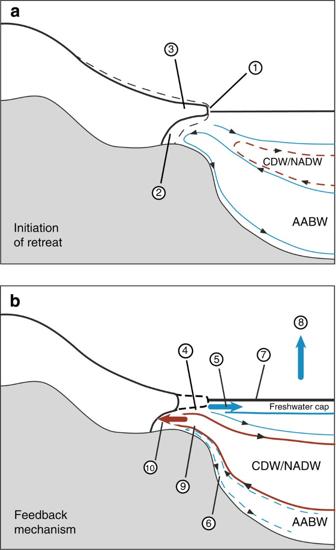Figure 7: A positive ice-ocean feedback mechanism for Antarctica. (a) Schematic representation of the AIS and ocean circulation at the LGM. 1: LGM ice sheet at continental shelf edge. 2: Slow thinning and grounding-line retreat. 3: Establishment/growth of ice shelf. (b) The positive feedback mechanism that allows a rapid sea-level contribution from Antarctica, based on inferences from proxy data (Fig. 5) and modelled atmospheric and oceanic temperature anomalies (Fig. 6). 4: Rapid weakening of SO overturning due to abrupt Atlantic Meridional Overturning Circulation (AMOC) recovery. 5: Freshening of ocean surface. 6: Reduced AABW formation. 7: Expansion/thickening of sea ice. 8: Atmospheric cooling (Antarctic Cold Reversal (ACR)). 9: Incursion of Circumpolar Deep Water (CDW) onto shelf. 10: Rapid thermal erosion at grounding line. In the absence of other stabilizing factors such as gravitational effects or grounding-line sedimentation, this meltwater maintains the stratification and the positive ice-ocean feedback. Full size image Figure 7: A positive ice-ocean feedback mechanism for Antarctica. ( a ) Schematic representation of the AIS and ocean circulation at the LGM. 1: LGM ice sheet at continental shelf edge. 2: Slow thinning and grounding-line retreat. 3: Establishment/growth of ice shelf. ( b ) The positive feedback mechanism that allows a rapid sea-level contribution from Antarctica, based on inferences from proxy data ( Fig. 5 ) and modelled atmospheric and oceanic temperature anomalies ( Fig. 6 ). 4: Rapid weakening of SO overturning due to abrupt Atlantic Meridional Overturning Circulation (AMOC) recovery. 5: Freshening of ocean surface. 6: Reduced AABW formation. 7: Expansion/thickening of sea ice. 8: Atmospheric cooling (Antarctic Cold Reversal (ACR)). 9: Incursion of Circumpolar Deep Water (CDW) onto shelf. 10: Rapid thermal erosion at grounding line. In the absence of other stabilizing factors such as gravitational effects or grounding-line sedimentation, this meltwater maintains the stratification and the positive ice-ocean feedback. Full size image This is not the case, however, for rapid subsurface warming events at 17 ka BP (0.028 Sv) and 11.8 ka BP (0.05 Sv), implying a secondary control. We propose that ice-sheet configuration is the critical second component. At 17 ka BP, the modelled AIS is not yet undergoing retreat and is insensitive to all of the applied ocean forcing combinations ( Fig. 3a ) due to its excess thickness above flotation at this time. At 11.8 ka BP, the ice-sheet responses in the FWF and NFW experiments are very different from one another, despite identical subsurface ocean warming. Enhanced discharge occurs under the NFW scenarios ( Fig. 3d ) because of the greater volume of grounded ice in the marine embayments compared with under FWF scenarios at this time ( Fig. 3a ). Thus, for the ice-ocean feedback to operate, we conclude that the ice sheet must be close to flotation in its marine sectors, but with a critical volume of ice still present in the marine basins. If these conditions are not met, the rate of mass loss will be insufficient to maintain oceanic stratification and the positive feedback will not occur. Recent observations show that the high-latitude Southern Ocean is becoming increasingly stratified due to freshening of its surface [25] , [26] . Future implications of this change, in terms of its effect on the AIS, can be assessed by comparison with periods of the recent past when similar oceanic conditions occurred. Here we have shown that the retreating LGM AIS had sufficient ice volume excess above present day (c. 14.5 m) to substantially contribute to MWP1A, when GMSL rose by 14–18 m in ~350 years [6] . This contribution reaches a maximum only when the effects of an abrupt reduction in high-latitude Southern Ocean overturning are included. Under such circumstances, rates of nearly 0.7 m per century s.l.e. are predicted at the time of MWP1A. Without this oceanic stratification, however, predicted mass loss from the ensemble mean amounts to ~0.3 m per century s.l.e. We propose that this change in Southern Ocean ventilation may have occurred as a consequence of the abrupt resumption of the Atlantic Meridional Overturning Circulation following H1, producing high-latitude subsurface warming that amplified the response of the already retreating ice sheet. Irrespective of the mechanism that may have initiated abrupt changes in Southern Ocean circulation, our results suggest that enhanced oceanic stratification may be a precursor for a positive ice-ocean feedback that under certain conditions could accelerate the retreat of marine-based sectors of the AIS. The ice-sheet model We used the Parallel Ice Sheet Model [27] to investigate decay of the AIS through Termination 1. Our experimental ensemble was implemented at 15 km resolution to allow computational tractability for large numbers of experiments. Building on previously established parameterizations [13] , [28] , we ran ~250 new simulations, primarily exploring a range of basal traction values and ice-flow enhancement factors, to achieve the closest possible fit to ice-sheet elevations inferred from continental ice cores and a lateral extent compiled from many marine surveys over recent decades [18] . The parameterization that produces our best fit is shown in Supplementary Table 1 . Parallel Ice Sheet Model (PISM) uses a combined stress balance approach that superposes velocity solutions of the two shallow approximations for sheet flow shallow ice approximation (SIA) and shelf flow shallow shelf approximation (SSA) across the entire model domain. This approach allows sheet and shelf flow to be treated in a consistent manner, and provides a valid approximation of the transition zone between grounded and floating ice [29] . Compared with grounding-line positions from semi-analytical calculations [30] , such as employed in the Marine Ice Sheet Model Intercomparison Project intercomparison [31] , the performance of PISM, and many other finite-difference ice-sheet models, is resolution dependent. The consequence of this is that fluxes across the grounding line may not be accurately represented, leading to grounding-line migration rates that underestimate those expected on theoretical grounds. This problem is exacerbated at shorter timescales, but may be mitigated to some extent by adopting a tuning methodology that reproduces more than one known grounding-line position. In our study, we fit to both LGM and present-day grounding lines. As ice shelves leave little record in geological archives, their probable LGM extents are unconstrained. Although we do not show them, shelves are nonetheless included in our simulations on the basis that they exert a buttressing effect on upstream grounded ice. A novelty of our study compared with previous simulations [3] , [28] is our implementation of a time-dependent basal substrate rheology. In this scheme, meltwater generated at the ice-sheet bed by geothermal, frictional and strain heating saturates, and therefore weakens the subglacial till layer. The reduced basal traction allows grounded ice to accelerate [32] , which in turn leads to dynamic thinning, a reduction in driving stress and ultimately the cessation of fast flow. Diffusive flow from upstream, coupled with local surface mass balance, subsequently allow the thinned ice stream to thicken, increasing driving stresses at the bed and eventually allowing reactivation of the ice stream (see Supplementary Movie 1 ). This cyclic behaviour [33] mimics ice-stream flow switching currently observed in AIS [34] , as well as being inferred from geological archives for past behaviour [35] . As the episodic behaviour of simulated ice streams arises during periods of ice-sheet stability (for example, before T1) as well as during periods of imbalance, it is not attributable to external (that is, environmental) forcings, but emerges from internal glaciological feedbacks. Glacio-isostatic loading of the underlying bedrock is an important component of our simulation, enabling the evolving ice-sheet geometry to effect changes in bed elevation according to the change in magnitude of the load and the viscosity of the underlying mantle. By consequence, changes in crustal load directly affect relative sea level as felt by the simulated ice sheet, providing a feedback that influences ice-sheet dynamics and extent. In PISM, the viscoelastic deformable Earth model employed combines a layered elastic spherical Earth with a viscous half-space overlain by an elastic plate lithosphere [36] . This model adapts a previous local model [37] for use in continental-scale ice-sheet simulations. It makes use of a novel numerical strategy that employs the fast Fourier transform to reproduce many of the key features of spherical, layered, self-gravitating viscoelastic Earth models, but with considerably reduced computational expense. By implementing a new mathematical formulation for the half-space model, this approach improves on the elastic plate lithosphere with relaxing asthenosphere model typically used in ice-sheet models, and produces smaller numerical errors than other Earth models. PISM does not, however, implement a gravitationally self-consistent sea-level model. Two components of this problem exist. First, short-term (<500 years) variations in ice mass lead to changes in the gravitational pull of neighbouring oceans and thus changes in relative sea level at the ice-sheet margin [38] . Second, over longer timescales the viscous response of the upper mantle and crust produce a redistribution of (bedrock) mass that also affects the gravitational pull on ocean water [39] . Together, these two effects may locally modify eustatic sea level by several metres, which under some scenarios may be sufficient to stabilize or slow the retreat of marine-based ice sheets [38] , [39] , or in the case of a growing ice-sheet, may lead to locally increased sea level and therefore slow the advance of grounding lines [40] . By neglecting these effects in our simulations, we implicitly smooth out any grounding-line migrations that might occur in response to small (<5 m) changes in sea level. However, in our ensemble approach, we use three different sea-level curves that at any given time vary by up to 10 m during the LGM to Holocene period. Thus, by considering our findings in terms of the ensemble mean, we directly capture any probable variability in ice-sheet response that may arise from sea-level changes of up to 10 m. The earth system model To specifically investigate the mechanisms that may have either induced or prevented rapid ice-sheet retreat and the generation of an Antarctic meltwater pulse, we used a range of sea-level and ocean-heat forcings. Of the latter, two time series forcings were generated from zonally averaged subsurface (485–700 m depth) ocean temperatures from transient deglacial simulations using the Earth System model LOVECLIM [11] . The two forcings differ only in that one incorporates a Southern Ocean meltwater pulse between 14.4 and 12.4 ka BP, and the other does not. Thus, differences in modelled ice sheet response between experiments using these two forcings arise purely as a consequence of the presence or absence of the prescribed freshwater input. In the experiment that incorporates the Southern Ocean meltwater pulse, a freshwater flux is added over the Southern Ocean between 14.4 and 12.4 ka B.P. An initial flux of 0.15 Sv is added for 1,000 years after which the input decreases linearly to 0 over the next 1,000 years. If directly translated into s.l.e., the freshwater flux added during MWP1A (14.4–14 ka BP) equates to 5.3 m sea-level rise. There are however several caveats. First, although the total Antarctic Bottom Water formation rate is well captured by the Earth System model, the AABW circulation is represented as a broad slow downslope flow, while in observations there is evidence of rapid confined flows within abyssal canyons off the continental slope. Second, melting of ice shelves would lead to additional freshwater input into the Southern Ocean but without raising sea level. Third, enhanced freshwater flux over the Southern Ocean could also be obtained by increased precipitation and/or reduced evaporation. For example, the 0.15 Sv would be equivalent to an additional 0.1 m per year precipitation over the Southern Ocean (75–50 S, calculated with the ocean area only). Ice-sheet model inputs and environmental forcing data We use the newest compilations of Antarctic bedrock topography [12] and surface mass balance [41] . The transient simulations also require time-dependent environmental forcings to most accurately reproduce changing conditions through the glacial termination. Air-temperature changes are prescribed according to the EPICA Dome C oxygen isotope record, using the EDC3 timescale [19] . Precipitation changes are implemented according to a temperature-dependent exponential function [2] , in which cooler air leads to a reduction in moisture-carrying capacity and hence a drier atmosphere. Sea-level changes are prescribed according to three recent interpretations of GMSL [6] , [7] , [8] ( Supplementary Fig. 1a ). Ocean heat fluxes are based on a global δ 18 O stack [9] , a Southern-Ocean δ 18 O record [10] and on two zonally averaged mid-depth temperature fields from LOVECLIM [11] ( Supplementary Fig. 1b ). Although the global δ 18 O stack [9] does not separate changes in oceanic temperature and changes in sea level, this and other similar records [42] have been employed previously to drive AIS simulations [3] , [43] and so is used here for completeness and to aid comparison with these (and other) models. As a direct translation of benthic δ 18 O values into ice-shelf basal melt rates is difficult, due to the combined complexities of converting isotopic values to ocean temperatures and of calculating melt rates from ‘mean’ ocean temperatures, we scaled all of our ocean heat time-series data to a melt rate range (0 to −20 m per year) that yielded both LGM and present-day ice-sheet extents that were most consistent with empirically determined grounding-line locations for these time periods. This range of melt rates is well within those currently experienced around Antarctica, although in some cases basal melt is thought to locally exceed 100 m per year in some areas [44] . One advantage of scaling the ocean forcing to reproduce two end-member states (LGM and present) is that the absolute magnitude of the imposed melt rate becomes less important. Simulated deglacial changes arise simply from the relative variation in rate-of-change of the applied forcing, irrespective of the absolute magnitude. Nevertheless, in the most extreme subsurface warming event simulated at the time of MWP1A in the Earth System Model (0.5–1 C), our scaling gives an equivalent melt-rate increase of ~10 m per year, a value that is within the range of those based on observational data from modern Antarctic ice shelves [45] , [46] . We acknowledge, however, that there is considerable uncertainty in the relationship between ocean temperature and ice-shelf melt, and that this is an area of considerable current research [47] . Lower melt rates reduce the magnitude, but not the timing, of our modelled rates of ice loss, and result in transient ice-sheet configurations that fit less well with observations. All of our environmental forcings are implemented uniformly across the domain and hence do not account for spatial differences in their timing or magnitude. Modelling approach All simulations are initialized from a spun-up present-day configuration AIS. The spin-up procedure involves an initial 100-year smoothing run, in which the model uses the primary input data directly, allowing the ice sheet to evolve by internal deformation only. This removes any steep gradients or inconsistencies in the input ice thickness data. From the outputs of this short run, a 50-kyr run is initialized that holds the ice-sheet geometry fixed but allows ice and bedrock temperature gradients to evolve to equilibrium. The final phase of experimentation employs a 30-kyr spinup before the 20-kyr T1 period of interest, during which full model physics are employed (bedrock loading, flow by sliding, as well as creep, evolution of basal meltwater and substrate rheology) and the ice sheet is allowed to evolve in response to imposed sea level, ocean heat, air temperature and precipitation perturbations. For each of our 250 simulations, model outputs were generated at 100-year intervals through the 50-kyr run, and were assessed against eight discrete criteria compiled from empirical interpretations of both temporal and spatial ice sheet evolution during T1 (see ‘Evaluation Criteria’). Progressive refinement of model fit was achieved by manual tuning of model parameters. Once a preferred parameter set had been achieved, a set of 12 experiments (representing the combination of three sea-level and four ocean heat forcings) was run. Evaluation criteria Several recent studies have attempted to gauge the closeness of fit of their results to empirical constraints by quantifying mismatches between the two [28] , [48] , [49] . In most cases, this amounts to comparing, for example, modelled ice elevations with those determined for periods such as the LGM from surface exposure dating (SED). Although this appears in principal to be a robust approach to understanding uncertainty in model outcomes, the validity of this seemingly objective analysis is predicated on the correct interpretation of the features from which the numerical constraints are derived. Recently, the assumption that surface exposure dates reflect the true former elevation of the LGM ice-sheet surface in Antarctica has been questioned [17] , [50] . These arguments are made on the basis that cold-based ice may have overlain SED sample sites, and left little geomorphological signature. Indeed, modelled temperature fields in LGM Antarctic glaciers such as Byrd Glacier highlight exactly this problem (ref. 13 and Fig. 2b therein), with warm-based ice restricted to the floor and lowest valley sides of the glacier trunk and cold-based ice occurring higher up. To avoid such problems, we adopt an approach that considers not only the geometry of the ice mass at a given point in time but also attempts to match our modelled behaviour to transient changes indicated by the collected body of empirical data. Specifically, we use primarily model-based inferences from ice cores in the interior of both East and West Antarctica to define the thinning or thickening pattern of each ice sheet through the last Termination ( Supplementary Table 2 ). Although sparse, these ice-core data are internally consistent in indicating a thinning of 100–120 m in central East Antarctica, and a thickening of 200–400 m in West Antarctica and in coastal areas ( Fig. 1 ). An additional, although less well constrained, check on our modelled ice-sheet evolution comes from measured uplift rates across Antarctica [51] , which provide an order-of-magnitude measure of ongoing glacio-isostatic adjustment to LGM loading. Marine geological data provide both temporal and spatial constraint on the growth and decay of the LGM ice sheet, generally indicating expansion to the continental shelf edge at LGM [18] followed by earliest retreat in the outer Weddell Sea embayment [52] and along the Antarctic Peninsula [53] . On this basis, outputs from each simulation were assessed against the following temporal and spatial constraints (in order of importance, based on area covered): (1) lateral extent at LGM reached almost to the continental shelf edge around the entire continent [18] ; (2) ice surface elevations in interior East Antarctica lowered by 100–150 m at LGM [19] , [54] ; (3) ice surface elevations in West Antarctica rose by 200–400 m at LGM [55] , [56] ; (4) grounded ice in the Ross Sea was fed from both East and West Antarctica, and was confluent around 180 longitude [57] ; (5) retreat from LGM extent began earliest in the Antarctic Peninsula [58] ; (6) retreat of the East Antarctic Ice Sheet started earliest in the Amery Trough, and later elsewhere [59] ; (7) ice in the western Ross Sea flowed around Ross Island and into McMurdo Sound, where it remained stable until ~13 ka BP (ref. 60 ); and (8) coastal parts of WAIS may have thickened during T1 and into the Holocene [61] . Finally, the geometry and surface velocities of grounded ice at the end of the run were compared with values from the most recent continent-wide syntheses of present-day ice thickness and velocity [12] , [62] . We consider these eight criteria a robust framework for model evaluation, but recognize that the use of other constraints (such as terrestrial SED data) would result in a slightly thinner ice sheet than the one we simulate. Quantifying the reliability of such geological proxies therefore remains an important area for future research. How to cite this article : Golledge, N. R. et al . Antarctic contribution to meltwater pulse 1A from reduced Southern Ocean overturning. Nat. Commun. 5:5107 doi: 10.1038/ncomms6107 (2014).